Questioning whether IgM Fc receptor (FcµR) is expressed by innate immune cells 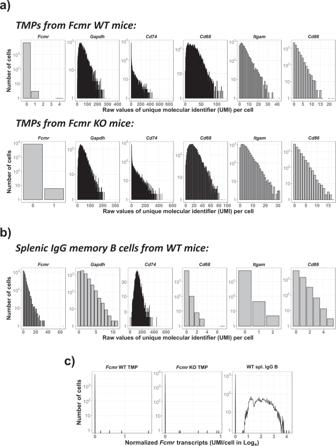Fig. 1: Gene detection histogram. a,bRaw values for the number of cells and the number of transcript reads (or unique molecular identifier; UMI) of the indicated genes in tumor-associated mononuclear phagocytes (TMPs) from C57BL/6FcmrWT (upper) and KO (lower) mice (a) and IgG memory B cells from C57BL/6 WT spleen (b), are plotted ony-axes andx-axes, respectively.cDensity curves of normalized UMIs forFcmrtranscripts in TMPs fromFcmrWT and KO mice and from WT splenic IgG B cells. The TMP data1were derived from GSE130287 and the IgG B cell data5from our scRNAseq analysis GSE140133. Note different scales of thex-axis for each gene. 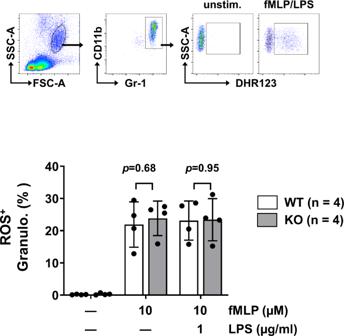Fig. 2: Production of reactive oxygen species (ROS) by granulocytes. Blood granulocytes from ourFcmrKO and WT C57BL/6 female mice of 8–12 weeks of age were loaded with 10 µM dihydrorhodamine 123 (DHR123), stimulated with or without 10 µMN-formyl-methionine-leucine-phenylalanine (fMLP) in the presence or absence of lipopolysaccharide (LPS; 1 µg/ml), and stained with PE-labeled Gr-1 and PE/Cy7-labeled CD11b mAbs, before lysis of erythrocytes and flow cytometric analysis. Top: Gating strategy for DHR123+Gr-1+CD11b+ROS-producing granulocytes. Bottom: Results are shown in mean ± 1 SD,n= 4Pvalues were calculated with an unpaired Studentt-test and a two-tailedPvalue of <0.05 was statistically significant. Note comparable ROS production between ourFcmrKO and WT mice, distinct from enhanced ROS production by theirFcmrKO granulocytes6. Single cell analyses The scRNAseq data of TMPs (GSE130287) from Fcmr WT and KO C57BL/6 mice [1] and splenic IgG memory B cells (GSE140133) from antigen-immunized WT C57BL/6 mice [5] , which are publicly available (see their repositories below), were reexamined as follows. R package Seurat v4.0.5 [11] was used to read deposited data sets. Raw count matrices were subject to quality control based on: (i) the number of cells where a gene was detected, (ii) the number of genes detected per cell, and (iii) the frequency of UMIs associated with mitochondrial genes. The final filtered matrices contained 16,112 genes and 14,352 cells (6352 Fcmr WT and 8000 Fcmr KO mice) for TMPs and 13,072 genes and 5436 cells for IgG B cells. Seurats LogNormalize-method with default settings was used to normalize UMI counts. Analysis of ROS production For ROS production, blood was collected from the submandibular vein of Fcmr WT and KO C57BL/6 female mice of 8–12 weeks by needle puncture in heparinized microfuge tubes. Twenty microliter of blood were mixed with 180 µl of 10 µM dihydrorhodamine 123 (DHR123; Marker Gene Technologies) in the absence or presence of 10 µM N- formyl-methionine-leucine-phenylalanine (fMLP) alone or along with lipopolysaccharide (LPS; Sigma) in DMEM/2% FCS in 96-well flat-bottom plates. After 30 min under 5% CO 2 at 37 °C, cells were washed with FACS buffer (PBS/2% FCS/0.1% NaN 3 ) and stained with PE-labeled GR-1 mAb (clone RB6-8C5) at 0.5 µg/ml and PE/Cy7-labed CD11b mAb (clone M1/70; eBioscience) at 0.67 µg/ml on ice for 20 min, before lysis of erythrocytes with 1 ml of Fix/Lysis buffer (PBS/1% formalin/0.07% saponin) on ice for 10 min. After washing, cells were resuspended in FACS buffer and granulocytes were first gated by high FSC and high SSC characteristics and then by positive for both Gr-1 and CD11b by Accuri C6 Flow Cytometer (BD). DHR123 + Gr-1 + CD11b + cells were defined as ROS-producing granulocytes. Approximately 50,000–70,000 cell events were acquired and analyzed with FlowJo software (BD). On average 5% of total blood nucleated cells were granulocytes for both groups of mice. Data comparison was performed by unpaired Student t- test (GraphPad Prism 9) and a two-tailed P value of <0.05 was defined as statistically significant. All studies involving animals were conducted with and after approval of the Landesamt für Gesundheit und Soziales (Lageso) and University of Alabama at Birmingham Institutional Animal Care and Use Committee (IACUC-09195). Reporting summary Further information on research design is available in the Nature Research Reporting Summary linked to this article.